Deficient angiogenesis in redox-dead Cys17Ser PKARIα knock-in mice Angiogenesis is essential for tissue development, wound healing and tissue perfusion, with its dysregulation linked to tumorigenesis, rheumatoid arthritis and heart disease. Here we show that pro-angiogenic stimuli couple to NADPH oxidase-dependent generation of oxidants that catalyse an activating intermolecular-disulphide between regulatory-RIα subunits of protein kinase A (PKA), which stimulates PKA-dependent ERK signalling. This is crucial to blood vessel growth as ‘redox-dead’ Cys17Ser RIα knock-in mice fully resistant to PKA disulphide-activation have deficient angiogenesis in models of hind limb ischaemia and tumour-implant growth. Disulphide-activation of PKA represents a new therapeutic target in diseases with aberrant angiogenesis. Angiogenesis is a pivotal process in tissue development and maintenance, as well as wound healing and repair. Inadequate angiogenesis resulting in under-perfusion of tissues mediates many pathologies including peripheral vascular and ischaemic heart disease [1] . Conversely, over-angiogenesis is a common feature of prevalent diseases such as cancer, rheumatoid arthritis and macular degeneration [2] . Growth factors which trigger angiogenic signalling also commonly couple to oxidase activation [3] , [4] . Indeed, vascular endothelial growth factor (VEGF), a potent inducer of endothelial cell migration and angiogenesis couples to oxidant production required for downstream signalling [5] , [6] . An essential role for oxidants is supported by antioxidant interventions blocking VEGF- or hypoxia-induced angiogenesis [7] , [8] . Several studies have identified nicotinamide adenine dinucleotide phosphate-oxidase (Nox) enzymes as a major source of oxidants required for angiogenesis [9] , [10] , [11] . Although oxidase enzymes mediate angiogenesis, little is known about the molecular targets that sense and transduce the growth-stimulating ‘oxidant signal’. Previously we showed the regulatory-RIα subunit of protein kinase A (PKA) can sense oxidants and transduce them into phosphorylation-mediated signalling [12] , [13] . This is potentially pertinent to angiogenesis as PKA is a widely-appreciated mediator of vessel growth [14] , [15] . Consequently, we investigated whether PKARIα oxidation is an essential step in the angiogenic pathway. The treatment of endothelial cells or aortic vessels with VEGF induced growth factor signalling and an angiogenic phenotype that was dependent on PKARI oxidation. These findings were physiologically translatable as transgenic mice unable to undergo PKARI oxidation had deficient vessel growth following hind-limb ischaemia or tumour implantation. VEGF induces signalling via PKARI oxidation Treatment of bovine aortic endothelial cells (BAECs) with VEGF induced canonical angiogenic signalling, namely phospho-activation of extracellular-signal-regulated kinase (ERK) and its downstream target cAMP response element-binding protein (CREB) ( Supplementary Fig. 1a ). ERK phospho-activation was also independently induced by hydrogen peroxide (H 2 O 2 ) treatment, in line with VEGF-induced oxidant production being an integral component of growth factor signalling ( Fig. 1a ). Consistent with our past studies [12] , [13] , we found that H 2 O 2 - or VEGF-induced oxidant formation oxidized PKARIα to a disulphide state ( Fig. 1a ). This disulphide in PKARIα enhances its affinity for A-kinase anchor proteins (AKAPs), serving to target the kinase to substrates it phosphorylates [12] , [16] . In addition to VEGF, the treatment of BAECs with insulin also induced PKARI oxidation ( Supplementary Fig. 1b ), suggesting a common mechanism may exist between receptor tyrosine kinases (RTKs) to induce oxidant formation. 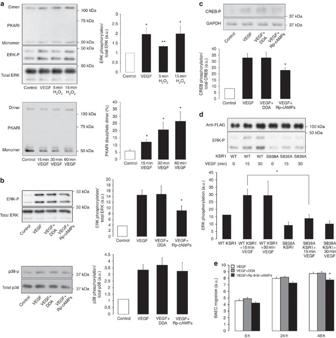Figure 1: VEGF induces growth factor signalling that is dependent on PKARIα oxidation. (a) PKARIα disulphide dimerization increased in a concentration-dependent manner in BAECs treated with either H2O2or VEGF (n=3). In addition, H2O2also induced a concentration-dependent increase in ERK phosphorylation, mimicking the effects of VEGF on growth factor signalling (n=3). (b) Increased ERK phosphorylation in BAECs stimulated with VEGF was attenuated by the PKA selective inhibitor Rp-8-Br-cAMPs (Rp-cAMPs) but not the adenylate cyclase inhibitor DDA (n=5). Neither inhibitor modulated VEGF-stimulated p38 mitogen-activated protein kinase phosphorylation. (c) The phosphorylation of CREB in BAECs stimulated by VEGF was attenuated by the PKA inhibitor Rp-8-Br-cAMPs (Rp-cAMPs) but not the adenylate cyclase inhibitor DDA (n=5). (d) Expression of S838A mutated KSR1 decreased VEGF-dependent ERK phosphorylation compared with WT (n=3) (e) Migration of BAEC by VEGF was partially attenuated by the PKA-specific inhibitor Rp-8-Br-cAMPs but not the adenylate cyclase inhibitor DDA (n=3). Data are shown as the mean±s.e.m. *P<0.05, **P<0.01 determined byt-test. Figure 1: VEGF induces growth factor signalling that is dependent on PKARIα oxidation. ( a ) PKARIα disulphide dimerization increased in a concentration-dependent manner in BAECs treated with either H 2 O 2 or VEGF ( n =3). In addition, H 2 O 2 also induced a concentration-dependent increase in ERK phosphorylation, mimicking the effects of VEGF on growth factor signalling ( n =3). ( b ) Increased ERK phosphorylation in BAECs stimulated with VEGF was attenuated by the PKA selective inhibitor Rp-8-Br-cAMPs (Rp-cAMPs) but not the adenylate cyclase inhibitor DDA ( n =5). Neither inhibitor modulated VEGF-stimulated p38 mitogen-activated protein kinase phosphorylation. ( c ) The phosphorylation of CREB in BAECs stimulated by VEGF was attenuated by the PKA inhibitor Rp-8-Br-cAMPs (Rp-cAMPs) but not the adenylate cyclase inhibitor DDA ( n =5). ( d ) Expression of S838A mutated KSR1 decreased VEGF-dependent ERK phosphorylation compared with WT ( n =3) ( e ) Migration of BAEC by VEGF was partially attenuated by the PKA-specific inhibitor Rp-8-Br-cAMPs but not the adenylate cyclase inhibitor DDA ( n =3). Data are shown as the mean±s.e.m. * P <0.05, ** P <0.01 determined by t -test. Full size image Following the novel observation that VEGF triggered RIα oxidation we examined its potential impact on downstream growth factor signalling. Phosphorylation of ERK induced by VEGF was substantially attenuated by the PKA inhibitor 8-Bromo-2′-monobutyryladenosine-3′, 5′-cyclic monophosphorothioate, Rp-isomer (Rp-8-Br-cAMPS). However, VEGF-induced activation of ERK was insensitive to the adenylate cyclase inhibitor 2′, 5′-dideoxyadenosine (DDA, Fig. 1b ). This is consistent with VEGF-induced activation of PKA being mediated directly by RIα oxidation, and not by the classical mechanism involving adenylate cyclase activation to generate cAMP. In contrast to ERK, VEGF-induced phospho-activation of p38 mitogen-activated protein kinase was unaffected by either inhibitor. A key downstream target of PKA and ERK crucial to angiogenesis, namely CREB was phosphorylated in response to VEGF and again was blocked by the PKA inhibitor Rp-8-Br-cAMPS, but not by adenylate cyclase inhibition ( Fig. 1c ). A role for PKARIα in angiogenic signalling is supported by studies showing that PKA and ERK form a signalling complex [17] . Here we also observed using immunofluorescence a pool of PKARIα basally co-localized with ERK in BAECs ( Supplementary Fig. 1c ). Complementary immunoprecipitation studies corroborated that the catalytic subunit of PKA co-purified with ERK under basal conditions ( Supplementary Fig. 1d ). The ability of PKA to enhance ERK phosphorylation has been previously attributed to the phosphorylation of kinase suppressor of rat sarcoma (Ras) 1 (KSR1), which enhances signalling through the classic Ras/mitogen-activated protein kinase growth factor signalling pathway [17] , [18] . KSR1 is phosphorylated by PKA at Ser838, enhancing activation of ERK by growth factor stimulation. Consistent with this, a S838A KSR1 mutant that cannot be phosphorylated by PKA showed attenuated VEGF-dependent ERK activation ( Fig. 1f ). To further understand the regulation of PKA by VEGF in isolated BAECs, the antioxidants EUK-134 or N-acetylcysteine (NAC) were assessed ( Supplementary Fig. 1e ). Both antioxidants failed to prevent PKARI oxidation or ERK phosphorylation in response to VEGF. In fact the presence of NAC potentiated both these responses to VEGF. Furthermore, NAC alone was sufficient to promote PKARI oxidation and ERK phosphorylation. PKARI oxidation mediates vessel growth Next, we assessed whether PKARIα oxidation-induced signalling functionally impacted on the phenotypical pro-angiogenic migration of endothelial cells. VEGF-induced BAEC migration, and mirroring ERK and CREB phospho-stimulation were blocked by Rp-8-Br-cAMPs but not DDA ( Fig. 1g ). In addition to migration, increased endothelial cell proliferation is also required for vessel growth. Therefore, we monitored BAEC proliferation, which was also inhibited by Rp-8-Br-cAMPs but not DDA ( Supplementary Fig. 1f ). The evidence presented so far in support of PKARIα oxidation mediating growth factor-induced endothelial cell migration and proliferation is based solely on cell studies. To definitively establish whether PKARIα oxidation is important to angiogenesis in vivo , we generated a novel Cys17Ser PKARIα ‘redox-dead’ knock-in (KI) mouse line that cannot undergo disulphide-activation. The KI mouse had no obvious overt phenotype, with normal body weight, heart weight and haematological parameters compared with wild-type (WT) littermates ( Supplementary Fig. 2a,b ). In addition, classic activation of PKA by cAMP was unaffected by mutation of cysteine 17 to a serine residue, as forskolin induced the same pattern and intensity of PKA substrate phosphorylation in blood vessels from either genotype ( Supplementary Fig. 2c ). To ascertain whether KI mice had impaired angiogenesis, we compared them with WT littermate controls using a validated aortic-vessel sprouting assay [19] . VEGF-induced vessel sprouting was substantially impaired in the aorta from KI mice compared with WTs ( Fig. 2a ), illustrating the importance of PKARIα oxidation in angiogenesis and corroborating experiments in endothelial cells. In addition, VEGF clearly induces PKARIα oxidation in WT vessels that was fully abrogated in KIs as expected ( Fig. 2b, c ). Consistent with this, VEGF-induced ERK activation was present in the WT aorta but absent in the redox-dead mutants ( Fig. 2c ). Subsequent unbiased Affymetrix mRNA analysis reassuringly corroborated our findings, as VEGF treatment significantly upregulated ERK-stimulated genes in the WT (but not KI) aorta ( Supplementary Fig. 3 ). This mRNA analysis also highlighted a greater increase in cancer-associated gene expression in WT compared with the KI aorta stimulated with VEGF. As mRNA analysis was performed on intact blood vessels, the cell type responsible for the changes could not be defined. Therefore to assess if the endothelium was crucial to the ERK signalling triggered by VEGF, we compared intact blood vessels with those with the endothelium removed mechanically. Endothelium-denuded aortas showed a substantial loss in total ERK content together with impaired induction of phospho-ERK in response to VEGF compared with intact vessels ( Fig. 2d ). The loss in ERK phosphorylation in response to VEGF may be an indirect consequence of removing the endothelium. However, the fact that relatively little ERK is found in denuded vessels suggests a majority of ERK signalling is likely confined to the endothelium, where it contributes to growth factor signalling and angiogenesis. This is further substantiated by experiments comparing proliferation or migration of endothelial cells isolated from the aorta of WT or KI mice. The chemotactic migration of aortic endothelial cells from WT in response to VEGF was absent in KI mice, where it was even lower than in unstimulated cells isolated from the same animal ( Fig. 2e ). In addition aortic endothelial cells isolated from WT mice proliferated significantly faster than those from the KI ( Fig. 2e inset panel). 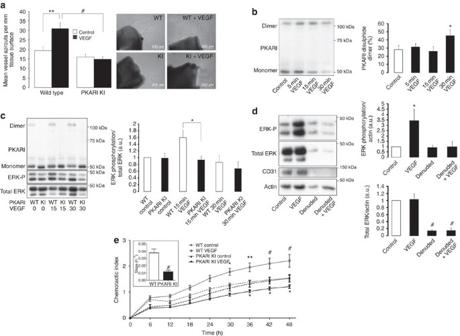Figure 2: Impaired aortic-vessel growth and ERK signalling in Cys17Ser PKARIα KI mice. (a) Vessel sprouting from cultured aorta was enhanced in those from wild-type mice treated with VEGF. This VEGF-dependent increase in aortic-vessel sprouting was absent in littermate KI PKARIα mice (n=8–12). (b) An increase in PKARIα disulphide dimerization was detected in cultured aorta following 30-min treatment with VEGF (n=7–8). (c) The oxidation of PKARIα was absent in aorta from KI mice as anticipated. Treatment of cultured wild-type aorta with VEGF increased ERK phosphorylation that was absent in littermate KIs (n=7–8). (d) Total ERK and its phosphorylation in response to VEGF was lost in endothelium-denuded aortic vessels (n=3–4). (e) The migration and proliferation (inset panel) of mouse aortic endothelial cells to VEGF in wild-type mice was impaired in those from KI animals (migrationn=5–7, proliferationn=6–8). Data are shown as the mean±s.e.m. *P<0.05, **P<0.01, #P<0.005 determined byt-test. Figure 2: Impaired aortic-vessel growth and ERK signalling in Cys17Ser PKARIα KI mice. ( a ) Vessel sprouting from cultured aorta was enhanced in those from wild-type mice treated with VEGF. This VEGF-dependent increase in aortic-vessel sprouting was absent in littermate KI PKARIα mice ( n =8–12). ( b ) An increase in PKARIα disulphide dimerization was detected in cultured aorta following 30-min treatment with VEGF ( n =7–8). ( c ) The oxidation of PKARIα was absent in aorta from KI mice as anticipated. Treatment of cultured wild-type aorta with VEGF increased ERK phosphorylation that was absent in littermate KIs ( n =7–8). ( d ) Total ERK and its phosphorylation in response to VEGF was lost in endothelium-denuded aortic vessels ( n =3–4). ( e ) The migration and proliferation (inset panel) of mouse aortic endothelial cells to VEGF in wild-type mice was impaired in those from KI animals (migration n =5–7, proliferation n =6–8). Data are shown as the mean±s.e.m. * P <0.05, ** P <0.01, # P <0.005 determined by t -test. Full size image Oxidation of PKARI regulates angiogenesis in vivo To further investigate the importance of RIα disulphide to angiogenesis in vivo , we implemented a hind-limb ischaemia and a tumour-implant model. Hind-limb ischaemia was induced by removing the femoral artery to severely limit distal blood flow ( Fig. 3a ). Over the subsequent 28 days there was a time-dependent return of blood flow due to angiogenesis, but this was significantly attenuated in KI mice compared with WTs. When implanted with breast cancer cells there was significantly less tumour growth in KI compared with WT mice ( Fig. 3b ). Immunofluorescent staining of blood vessels in tumour tissue using an antibody to the endothelial marker CD31 showed there was a deficit in vessel growth in those from PKARI KI mice compared with WTs ( Fig. 3c ). This provides robust evidence of a pivotal role for PKARIα oxidation in stimulating angiogenesis in vivo . 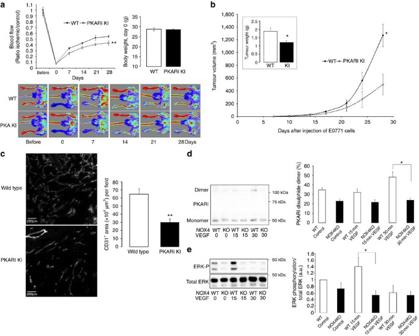Figure 3: Impaired angiogenesis in Cys17Ser PKARIα ‘redox-dead’ KI mice. (a)The removal of the femoral artery severely restricted blood flow within the hind limb of KI and littermate WTs as monitored using laser Doppler. Over the subsequent 28 days, there was a time-dependent return of blood flow to the hind limb of wild-types that was significantly attenuated in KI mice (n=6–7). (b) In mice injected with E0771 cells, there was a significant decrease in the growth and overall weight (inset panel) of tumours in KIs compared with WTs (n=5–7). (c) Less of the endothelial cell marker protein CD31 was observed in PKARI KI tumour tissue compared with WTs detected using immunofluorescence (n=4–5 tumours). (d) The oxidation of PKARI in cultured wild-type mouse aorta treated with VEGF was absent in aorta from littermate knockout Nox4 mice (n=8–11). (e) The enhanced phosphorylation of ERK in wild-type mouse aorta treated with VEGF was absent in aorta from littermate knock-out Nox4 mice (n=6–8). Data are shown as the mean±s.e.m. *P<0.05, **P<0.01 determined byt-test. Figure 3: Impaired angiogenesis in Cys17Ser PKARIα ‘redox-dead’ KI mice. ( a )The removal of the femoral artery severely restricted blood flow within the hind limb of KI and littermate WTs as monitored using laser Doppler. Over the subsequent 28 days, there was a time-dependent return of blood flow to the hind limb of wild-types that was significantly attenuated in KI mice ( n =6–7). ( b ) In mice injected with E0771 cells, there was a significant decrease in the growth and overall weight (inset panel) of tumours in KIs compared with WTs ( n =5–7). ( c ) Less of the endothelial cell marker protein CD31 was observed in PKARI KI tumour tissue compared with WTs detected using immunofluorescence ( n =4–5 tumours). ( d ) The oxidation of PKARI in cultured wild-type mouse aorta treated with VEGF was absent in aorta from littermate knockout Nox4 mice ( n =8–11). ( e ) The enhanced phosphorylation of ERK in wild-type mouse aorta treated with VEGF was absent in aorta from littermate knock-out Nox4 mice ( n =6–8). Data are shown as the mean±s.e.m. * P <0.05, ** P <0.01 determined by t -test. Full size image We sought to identify the molecular source of oxidants responsible for PKARIα oxidation. Recently three independent studies have specifically implicated Nox4 as an isozyme of NADPH oxidase that coupled to angiogenesis [9] , [10] , [11] . Consequently, we compared VEGF-induced RIα oxidation in the aorta from Nox4 knockout (KO) mice with littermate WTs, finding the former were substantially deficient ( Fig. 3d ). In contrast, PKARI in Nox4 KO mice could be oxidized by exogenously applied H 2 O 2 and was also classically activated by elevated cAMP. This is consistent with the deficient response of Nox4 KO to VEGF being specifically due to loss of this oxidase enzyme ( Supplementary Fig. 4a,b ). We also found that VEGF-induced ERK activation was deficient in Nox4 KO mice, which is in line with our observation that RIα oxidation was required for full phospho-activation of ERK ( Fig. 3e ). Our observations are also consistent with recent observations that Nox4 KO mice are deficient in their angiogenic response to the same hind-limb ischaemia implemented to RIα redox-dead mice [9] , [10] , [11] . Nox-derived oxidants can act as powerful mediators of growth factor signalling [10] , [11] , [20] . However, the targets of these oxidants and the mechanism by which they enhance vessel growth have remained elusive. In this study, we identified PKA as a target of oxidation that can transduce VEGF-dependent oxidant formation into pro-angiogenic signalling. The treatment of BAECs or isolated aortic vessels with VEGF resulted in disulphide dimerization of PKARI associated with its activation [12] . Once activated, oxidized PKA stimulated ERK, a principle mediator of growth factor signalling that couples with upregulation of genes involved in endothelial cell migration and proliferation [21] . It is likely that oxidized PKA activates ERK by directly phosphorylating the associated scaffold protein KSR1 to enhance throughput through the growth factor signalling pathway [17] . Although it is also conceivable that other PKA-dependent pathways may also contribute to the activation of ERK. Antioxidants failed to prevent VEGF-dependent BAEC PKARI disulphide oxidation or ERK phosphorylation. This failure of antioxidants to block oxidation of PKARI and consequent signalling is perhaps surprising to some, and an issue that warrants some detailed consideration. A prevalent idea has been that antioxidant molecules can react with oxidants and prevent them oxidizing their protein targets, which in this case are cysteine thiols in PKARI. This concept is the same, underlying antioxidants being therapeutic by preventing target oxidation (that is, damage). First, we should recognize that antioxidant therapy clinical trials have failed, and in some cases the intervention actually caused harm [22] , [23] , [24] . For example, in cancer where over-angiogenesis can occur, antioxidant trials have been stopped early because of increased mortality [24] , [25] . In this connection, it is notable that we found NAC potentiated pro-angiogenic PKARI and ERK signalling. Antioxidants are reductants, which by definition are electron donors, and so potentially may fuel oxidase enzymes to actually enhance oxidant generation and exacerbate target oxidation. NAC is also likely to react with oxidants to generate a disulphide derivative, which can potentially induce protein oxidation via thiol–disulphide exchange chemistry. Conversion from a reducing to an oxidizing form that induces protein oxidation has been demonstrated for the small thiol ‘antioxidant’ hydrogen sulphide [26] , [27] . Furthermore, many oxidants react faster with proteins than with antioxidants, so even when these small reducing molecules are used at high concentration they may not be effective in preventing target oxidation. Even if antioxidants effectively intercept oxidants, eventually they may become exhausted and, as mentioned, their oxidized end-products, which may induce protein oxidation, accumulate. Thus antioxidants are likely not as effective, in the context of blocking oxidant-induced signalling, as often they are simplistically anticipated to be. Therefore, while perhaps not intuitive, for the reasons discussed, we think our observation of NAC enhancing PKARI oxidation is not wholly unexpected from a mechanistic standpoint. Interestingly, in addition to VEGF the RTK ligand insulin is also able to induce PKARI oxidation. It may be that the RTKs couple to the same oxidase to induce signalling through protein oxidation. This is supported by evidence of insulin-induced angiogenesis through a Nox4-dependent mechanism [28] , [29] . The source of oxidants in VEGF-stimulated endothelial cells required for the oxidation of PKARI appears to be Nox4, as mice deficient in this oxidase lack the ability to undergo growth factor-dependent PKARI oxidation in isolated vessels. Although Nox4 is a known mediator of angiogenesis it still remains unclear how its activity is actually regulated by growth factors. One study suggests interaction of Nox4 with Rac1 stimulates oxidant generation that could drive acute oxidant signalling [30] . However this finding still remains to be confirmed. The emerging role of PKARI and Nox4 in vessel growth makes them potentially important drug targets, with their pharmacological inhibition having the potential to attenuate vessel growth in diseases such as cancer. The generation of a transgenic C42S PKARI KI mouse line that was engineered to be fully resistant to oxidation allowed us to definitively evaluate the role of PKA oxidation in regulating angiogenesis. To test the angiogenic potential of these mice, we utilized a hind-limb ischaemia and a tumour growth model, both of which are dependent on vessel growth. Loss in PKARI oxidation in PKARI KI mice significantly impaired blood vessel re-growth after hind-limb ischaemia and also reduced tumour growth and vascularization when compared with littermate WTs. Together, this provides a molecular mechanism for how growth factor-derived oxidants can mediate angiogenesis. Multiple cell-types involving numerous, complex signalling processes participate in new vessel formation, growth and maturation. A principal event in the early stages of vessel formation is the proliferation and chemotactic migration of endothelial cells in response to growth factor stimulation. In this study, we have identified the oxidation of PKA as a key event in endothelial cell growth factor signal transduction that mediates the cellular changes required for vessel growth. In endothelial cells isolated from the aorta of PKA KI mice, the migration induced by VEGF was not only absent, but was lower than in cells from the same animal basally without growth factor stimulation. This unexpected phenomenon suggests VEGF may mediate both pro-, as well as anti-angiogenic signalling. This is consistent with evidence that splice variants of VEGF can have opposing effects on vessel growth [31] , [32] . In this scenario, PKA in its oxidized form induces pro-angiogenic signalling that overrides the possible concomitant anti-angiogenic effects of VEGF to have a net increase in vessel growth. Overall, we conclude that PKARIα oxidation is a key event in VEGF-, tumour- and hind-limb ischaemia-induced angiogenesis. The oxidants that drive this signalling pathway that couples to ERK activation are derived in part from Nox4. Drugs that modulate the oxidative activation of PKARIα may have therapeutic potential in diseases with dysregulated angiogenesis. Western immunoblotting Western immunoblotting was carried out after protein separation by SDS–PAGE, with the addition of 100 mM maleimide in lysis buffer to alkylate thiols preventing disulphide exchange. Immunoblots were probed with primary antibodies to PKARI (1:1,000, BD Biosciences), PKAC (1:1,000, BD Biosciences), phospho (1:1,000, Thr202/Tyr204, Cell Signaling) and total ERK (1:1,000, Cell Signaling), phospho (1:1,000, Thr180/Tyr182, Cell Signaling) and total P38 (1:1,000, Cell Signaling), phospho (1:1,000, Ser133, Cell Signaling) and total CREB (1:1,000, Cell Signaling), PKA phospho-substrate (1:1,000, Cell Signaling) and anti-FLAG (1:1,000, Sigma). In addition horseradish peroxidase-linked secondary antibody (1:1,000, Cell Signaling) and enhanced chemiluminescence (ECL) reagent (Pierce) were used. Digitized immunoblots were quantitatively analysed using Gel-Pro Analyzer 3.1. The uncropped gel images are shown in Supplementary Figs 5 and 6 . PKARI oxidation status was determined as before by measuring the amount of this protein in the reduced monomeric and disulphide oxidized dimeric states and calculating the percentage oxidized [33] . Cell culture BAECs (Cell Applications, B304K-05) were cultured in Dulbecco's Modified Eagle Medium (DMEM, 31885-023 Invitrogen) supplemented with 10% foetal bovine serum (FBS, Invitrogen) and 1% penicillin–streptomycin (P/S). For experimental treatments, BAECs were grown until 80% confluent before being starved overnight in DMEM +1% P/S without FBS. Treatment of BAECs included 30-min incubation with 10 μM DDA or 100 μM Rp-8-Br-cAMP before addition and co-incubation with 50 ng ml −1 VEGF for 15 min. In separate experiments, serum-starved BAECs were treated with 100 μM EUK-134 or 0.5 mM NAC for 1 h before treatment with 50 ng ml −1 VEGF for 15 min. After treatment, media was removed and cells were immediately lysed into Laemmli sample buffer supplemented with 100 mM maleimide. Rapid lysis into alkylating agent was used to stabilize protein oxidation. In transfection experiments, C-terminal Flag-tagged KSR1 (Addgene, 25970) was expressed for 24 h before further treatment. Immunoprecipitation BAECs grown on six-well plates until 90% confluent were starved overnight. Cells were washed in phosphate-buffered saline (PBS) and then lysed into RIPA buffer and protease inhibitors (Roche, cOmplete protease inhibitor cocktail tablets).The supernatant from pelleted cell lysates was incubated overnight at 4 °C with 1 μl of primary antibody before the addition of A/G Sepharose beads (Santa Cruz). After 2 h incubation at 4 °C, the A/G Sepharose beads were washed three times with RIPA buffer. Immunoprecipitated proteins were then eluted from the Sepharose beads by addition of Laemmli sample buffer. Confocal microscopy Confocal microscopy was carried out using a Perkin Elmer spinning disk confocal microscope. BAECs were starved for 24 h in DMEM and 1% P/S before being fixed with 4% fresh paraformaldehyde for 15 min. After incubation, cells were washed three times and then permeabilized in 2 mg ml −1 saponin for 10 min before being blocked in 5% BSA for 1 h. After blocking, samples were washed three times and then incubated overnight at 4 °C with antibodies to ERK (1:200, Cell Signaling) and PKARI (1:40). BAEC migration assay Endothelial cell migration was determined using an Oris migration assay (Platypus Technologies) following the manufacturer’s instructions. In brief, cell seeding stoppers were securely placed into individual wells of a 96-well plate. To each well was added 100 μl of trypsinized BAECs in DMEM+10% FBS. After 24 h incubation at 37 °C in a cell culture incubator (95% O 2 /5% CO 2 ), the media in each well was replaced with DMEM supplemented with 1% P/S and FBS. After a further 24 h, the media in each well was replaced with DMEM containing 1% P/S and 1% FBS supplemented with 5-(and-6)-carboxyfluorescein diacetate, succinimidyl ester. After 25 min of incubation, the cell seeding stoppers were removed and the media in each well was replaced, either with DMEM containing 1% P/S and FBS or this media supplemented with 50 ng ml −1 VEGF, 50 ng ml −1 VEGF with 10 μM DDA or 50 ng ml −1 VEGF with 100 μM Rp-8-Br-cAMP. The number of cells migrated to the centre of each well was determined by attaching a detection mask to the cell culture plate and then measuring fluorescence at 6, 24 and 48 h using a Fluorescence plate reader (Fluostar omega, BMG labtech). BAEC proliferation assay Confluent BAECs where trypsinized in 0.05% trypsin-EDTA then re-suspended in DMEM+10% FBS. Suspended BAECs were counted and then seeded at a density of 2,500 cells per well on a 96-well E-plate (ACEA). Each well was then supplemented with DMEM to dilute the FBS to 5% and some were exposed to 10 μM DDA or 100 μM Rp-8-Br-cAMP. The cell index for each well was then measured over 48 h using the xCELLigence RTCA MP system (ACEA) at 37 °C in a cell culture incubator (95% O 2 /5% CO 2 ). The rate of cell proliferation was calculated from the gradient of each cell index by software provided by the manufacturer. Generation of KI C17S PKARI mice Mice constitutively expressing PKARI Cys17Ser were generated for us on a pure C57BL/6 background by TaconicArtemis. A targeting vector was constructed for murine Prkar1a by introducing the Cys17Ser mutation into exon 1 by site-directed mutagenesis and inserting an FRT-flanked neomycin selection marker (to allow for selection of transfected embryonic stem (ES) cells) close to the mutation to favour homologous recombination ( Supplementary Fig.7 ). Then screening by Southern blot was carried out to identify if homologous recombination had occurred followed by validation of the positive clones. ES cell transfection was then carried out followed by chimera generation. The chimeras were directly bred with an Flp deletor for the in vivo deletion of the selection marker. As the ES cells always go germline, chimeras can be directly bred to the deletor to obtain germline transmission and selection marker deletion at the same time. Mouse aortic endothelial cell isolation and analysis Crude endothelial cells were isolated from the mouse aorta. First, isolated vessels were canulated with a 24-gauge BD Angiocath and injected with 0.1% collagenase, followed by 5-min incubation at 37 °C. Endothelial cells were then flushed from vessels by injecting 2 ml of EGM-2MV media and repeating this 10 times. Endothelial cells were then further purified by labelling with CD31 (PE-CD31, eBioscience) and sorted by FACS aria II (BD) [34] . Once purified, endothelial cells were cultured with EGM-2MV media (Lonza) and passaged four times before analysis. In this study, endothelial cells were analysed in separate isolations from two WT and two PKARI KI mice. To analyse endothelial cell proliferation, isolated cells were seeded at a density of 15,000 cells per well onto a 16-well E-plate, and for migration 2,000 cells per well were seeded onto a transwell CIM-Plate 16 (ACEA Biosciences). When analysing proliferation, cells were maintained in EGM-2MV media, and for migration cells were first seeded in EBM-2 with 2% FBS, then prior to starting analysis serum starved for 18 h before addition of a lower chamber containing 5 ng ml −1 of VEGF. The migration and proliferation of isolated mouse endothelial cells was monitored using a RTCA DP Analyzer (ACEA Biosciences) following the manufacturer’s instructions. Haematological analysis Venous blood from WT or PKARI KI mice were analysed with a hand-held iSTAT analyser using EC8+ cartridges (Abbott Laboratories). Aortic sprouting assay Freshly isolated mouse aortic vessels were cleaned of fatty tissue and then rinsed in sterile PBS before being cut into ∼ 2 mm rings. Each ring was rinsed in fresh sterile PBS before being placed into individual wells on a 96-well plate pre-coated with basement membrane extract (60 μl per well, Trevigen). After 1-h incubation at 37 °C in a cell culture incubator (95% O 2 /5% CO 2 ), 100 μl of culture media (EBM-2, Lonza) containing 1% FBS, 1% P/S and supplemented with or without 50 ng ml −1 VEGF was carefully placed into each well. After 4-days incubation at 37 °C in a cell culture incubator, a further 200 μl of fresh culture media with the same supplementation was placed into each well. At 9 days, after aortic isolation the vessels were visualized using a Nikon eclipse ts100 microscope and then digitized. The quantity of sprouts and surface area of each aorta was determined using SigmaScan. Affymetrix analysis Freshly isolated mouse aortic vessels were cultured as stated above for sprouting assays in culture media (EBM-2) containing 1% FBS and 1% P/S for 24 h. After incubation, vessels were supplemented with fresh media with or without the addition of 50 ng ml −1 VEGF. After a further 24 h, vessels were snap-frozen in liquid nitrogen and mRNA extracted using a RNeasy Plus Universal Kit (Qiagen). About 50 ng of total RNA was processed using an Ovation WTA PicoSL V2 kit (NuGEN). About 5 μg of SPIA-amplified complementary DNA was fragmented and biotin-labelled using the Encore Biotin module (NuGEN), and hybridization cocktails prepared as recommended by NuGEN. Samples were hybridized to Mouse Gene 2.0 ST arrays using standard protocols as recommended by the manufacturer (Affymetrix). Arrays were scanned using GCS3000 scanner and the resulting image intensity (CEL) files were processed using the RMA-sketch algorithm in Expression Console software (Affymetrix), to generate normalized, background-corrected, summarized data files (CHP format). All chips passed basic data quality control checks as suggested by Affymetrix. Pathway analysis was performed independently by the core genomics facility under the guidance of Matthew Arno (Genomics Centre Manager) using pathway analysis (Thomson Reuters systems biology solutions). Microarray data have been deposited in the GEO repository under accession code GSE70216. Hind-limb ischaemia All procedures were performed in accordance with the Home Office Guidance on the Operation of the Animals (Scientific Procedures) Act 1986 in the United Kingdom. Hind-limb ischaemia (HLI) was performed in mice (male, 14–16 weeks of age) anaesthetized with 1.5% isoflurane in 0.5 l min −1 oxygen with pre- and post-operative analgesia (buprenorphine, 0.1 mg kg −1 of body weight) and placed on a heated blanket to maintain body temperature. The portion of the left femoral artery was exposed via 2-cm incision and two ligations were performed using eight nylon sutures, first distal to the origin of the profunda femoris artery and second proximal to the saphenous artery. The left femoral artery was then excised between the ligation sites and the skin was closed with non-continuous absorbable suture. Non-invasive laser Doppler imaging (MoorLDI2 model; Research Software 5.3, Moor Instruments Inc., Wilmington, USA) was used to assess hind-limb blood flow at baseline, and immediately after undergoing the HLI procedure with follow-up imaging performed 7, 14, 21 and 28 days after the HLI. The ratio of blood flow in ischaemic versus non-ischaemic limb was analysed from at least two high-quality images. Tumour growth All procedures were performed in accordance with the Home Office Guidance on the Operation of the Animals (Scientific Procedures) Act 1986 in the United Kingdom and were approved by the King’s College London Animal Welfare and Ethical Review Body. The E0771 spontaneous tumour cell line originally isolated from C57BL/6 mice (CH3 Biosystems) were cultured in RPMI 1640 medium supplemented with 10 mM HEPES, 10% FBS and 1% P/S. Before implantation, cells were trypsinised, re-suspended in PBS and counted using a haemocytometer. Each mouse (female, 12–14 weeks of age) was injected in the lower abdomen mammary fat pad with 5 × 10 5 E0771 cells and then closely monitored over a 24-h period. Tumour size was routinely measured using callipers and was not allowed to exceed 1.5 cm 3 . At 28 days, mice were euthanized followed by removal of tumours that were then weighted. Vessel imaging Excised tumours were frozen in liquid nitrogen-cooled isopentane. They were then embedded in optimal cutting temperature (OCT) compound and sectioned at −20 °C using a cryostat. Sections were fixed in acetone, blocked and immunostained using a fluorescently labelled CD31 antibody (1:200, Alexa Fluor 488 anti-mouse CD31 antibody clone MEC13.3, BioLegend). Immunostained sections were visualized using a Nikon eclipse ts100 fluorescence microscope, and images analysed for CD31 staining using ImageJ ( http://imagej.nih.gov/ij/ ). Treatment of aorta Excised aortas cleaned of fatty tissue were rinsed in sterile PBS within a cell culture hood. The aorta were then carefully cut into ∼ 2-mm rings. Each ring was rinsed in fresh sterile PBS before being placed into individual wells on a 96-well plate preloaded with 100 μl of DMEM+1% P/S. The aortic segments were then incubated overnight at 37 °C in a cell culture incubator (95% O 2 /5% CO 2 ). The following day, aortic segments were treated with or without 50 ng ml −1 VEGF for 15 min or 30 min before being snap-frozen in liquid nitrogen. In some experiments, the aorta where denuded by passing a 27 gauge needle through the vessel and then gently rotating eight times while submerged in PBS. Statistical analysis Results are presented as mean±s.e.m. Sample size required to achieve statistical significance was estimated using a power calculation based on past experience of anticipated differences between groups and group variance. Data from in vitro or cell-based studies were only excluded if there was a technical failure. No animals were excluded from the hind-limb ischaemia study, and one mouse was excluded from the tumour growth study because the implanted cells failed to grow. Differences between groups, in studies that were not blinded or randomized, were assessed using analysis of variance followed by a t -test. In addition, where more than two groups were compared, they were assessed using a Bonferroni correction. Differences were considered significant at the 95% confidence level. Accession codes. Microarray data have been deposited in the GEO repository under accession code GSE70216 . How to cite this article: Burgoyne, J. R. et al. Deficient angiogenesis in redox-dead Cys17Ser PKARIα knock-in mice. Nat. Commun. 6:7920 doi: 10.1038/ncomms8920 (2015).